Stimuli-responsive selection of target DNA sequences by synthetic bZIP peptides One of the strategies used by nature to regulate gene expression relies on the stimuli-controlled combination of DNA-binding proteins. This in turn determines the target-binding site within the genome, and thereby whether a particular gene is activated or repressed. Here we demonstrate how a designed basic region leucine zipper-based peptide can be directed towards two different DNA sequences depending on its dimerization arrangement. While the monomeric peptide is non-functional, a C-terminal metallo-dimer recognizes the natural ATF/CREB-binding site (5′-ATGA cg TCAT-3′), and a N-terminal disulphide dimer binds preferentially to the swapped sequence (5′-TCAT cg ATGA-3′). As the dimerization mode can be efficiently controlled by appropriate external reagents, it is possible to reversibly drive the peptide to either DNA site in response to such specific inputs. This represents the first example of a designed molecule that can bind to more than one specific DNA sequence depending on changes in its environment. The pattern of gene expression in a multicellular organism is determined by the action of defined extracellular cues and/or environmental signals that ensure the production of specific proteins only when and where needed. In most of the cases, these signals work by switching the activity of transcription factors (TFs), key gene regulatory proteins that promote the expression of selected genes by binding to relatively short stretches of specific regions of the DNA [1] , [2] . Among the different mechanisms used by nature to activate or inactivate TFs, those that affect their DNA-binding properties are particularly prominent [3] , [4] , [5] . In this context, it is well known that many TFs are unable to bind to their DNA targets by themselves and need to form cooperative multimeric complexes with other partners. This is a clever regulatory mechanism used by nature that allows the combinatorial interaction with a large number of sites using a relatively small set of monomeric transcription regulators [6] , [7] , [8] . For instance, the basic region leucine zipper (bZIP) family of DNA-binding proteins can bind DNA as homo- or heterodimers, and in this way recognize different DNA sites depending on the regulated combination of dimerization partners [9] , [10] . Over the last years there have been many reports on the design and preparation of short synthetic peptides capable of reproducing the basic DNA recognition properties of natural TFs [11] , [12] , [13] . Particularly relevant are those based on dimeric bZIP basic regions, in which the natural C/C-terminal leucine zipper is replaced by artificial dimerizers [14] , [15] , [16] , [17] . Some of these designs have gone even further and incorporate switchable elements that allow conditional off/on DNA binding by the application of external stimuli such as light or metal ions [18] , [19] , [20] , [21] , [22] . Despite advances in these and other switchable DNA binders [23] , [24] , designed systems capable of interacting with alternative DNA sites in an externally regulated manner are unknown. Herein we prove for the first time the concept of ‘site switchability’ in the DNA binding of synthetic systems, and demonstrate how a single bZIP-based peptide can be directed towards two different DNA sequences depending on its dimerization arrangement. As the dimerization can be controlled by the application of selected reagents, the methodology allows remote control of the DNA site selectivity. In addition to providing a simplified model of the natural mechanism of combinatorial DNA recognition, our work set the bases for future achievements on the stimuli-controlled differential expression of selected genes. The bZIP family of TFs is characterized by a C-terminal coiled-coil leucine zipper dimerization domain and a highly charged, N-terminal basic region, that mediates DNA binding [25] , [26] , [27] . In addition to the straightforward substitutions of the dimerization domain described before, the GCN4 bZIP-binding domain has inspired the development of a variety of synthetic, sequence-selective DNA-binding peptides [28] , [29] , [30] , [31] , [32] , [33] , [34] . Interestingly, although in all naturally occurring bZIP proteins the basic region is positioned N-terminal to the leucine zipper, Oakley and coworkers [35] showed that model ‘reverse’ bZIP peptides, in which the basic region of the bZIP factor GCN4 is placed C-terminal to its leucine zipper, can specifically bind to inverted DNA sites. Thus, while natural GCN4 C/C-terminal dimers specifically bind to ATF/CREB (5′-ATGA(c/g)TCAT-3′) or AP1 (5′-ATGA(c)TCAT-3′) sites, reversed N/N-terminal dimers bind to inverted 5′-TCAT(…)ATGA-3′ sites. Additionally, Morii et al . [36] had also previously described synthetic N-terminal dimers of GCN4 with selectivity towards the swapped-binding site. On these grounds, we envisioned that an appropriate dimerization of a GCN4 basic region through either its C- or the N-terminal side might allow to target two different sites by the same peptide unit. In addition, if the peptide is equipped with orthogonally responsive elements so that either dimerization can be triggered in response to different external stimuli, we would be in position to couple site selectivity to external inputs ( Fig. 1 ). The resulting system would, therefore, represent a simplified model of the combinatorial DNA recognition in natural TFs. Reversibility would be an additional and highly desirable property as it might endow site switchability. 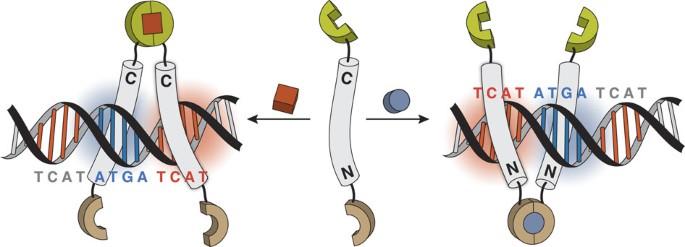Figure 1: Representation of a stimuli-responsive dimerization strategy for specific binding to two DNA sites. A modified peptide derived from the GCN4 TF contains orthogonal functionalities at both termini that in response to different stimuli (represented as a cube or a cylinder) result in alternative dimerization states with different DNA-binding preferences: 5′-ATGA(…)TCAT-3′ for the natural C/C-terminal dimer (left), or reversed 5′-TCAT(…)ATGA-3′ for the non-natural N/N-terminal dimer (right). Figure 1: Representation of a stimuli-responsive dimerization strategy for specific binding to two DNA sites. A modified peptide derived from the GCN4 TF contains orthogonal functionalities at both termini that in response to different stimuli (represented as a cube or a cylinder) result in alternative dimerization states with different DNA-binding preferences: 5′-ATGA(…)TCAT-3′ for the natural C/C-terminal dimer (left), or reversed 5′-TCAT(…)ATGA-3′ for the non-natural N/N-terminal dimer (right). Full size image Peptide design and synthesis Based on earlier reports by Schepartz and co-workers [17] , [37] on the use of metal-terpyridine complexes as dimerization elements for bZIP basic regions, we chose a terpyridine chelating ligand for the C-terminal end of the GCN4 basic region. This would allow promoting the dimerization by addition of a metal ion and formation of a stable metal complex with two terpyridine-tagged basic regions, while providing for reversibility. For the N-terminal dimerization, we selected a disulphide bond, as it could be easily implemented by introduction of a N-terminal cysteine residue. The disulphide bridge is sensitive to oxidizing or reducing conditions, and should be chemically orthogonal to the metal-mediated C-terminal dimerization. The starting point for our design is the truncated Asp226-Gln248 GCN4 basic region, which had been identified as the minimum length required for specific DNA binding [14] . This core sequence was extended with a cysteine residue at the C-terminus (introduced as trityl derivative) that would act as a nucleophilic handle for attachment of the terpyridine ligand. The N-terminal connection was engineered by adding a Cys–Gly linker to the Lys231 side chain, which was introduced as an Alloc-protected derivative to allow its selective deprotection on the solid-phase using palladium catalysis. The resulting linker is geometrically equivalent to the linker described by Morii et al . [36] in their studies of N-terminal covalent dimers of GCN4 basic regions ( Supplementary Fig. S1 ). In order to differentiate both thiols, the N-terminal Cys was introduced protected as Cys(tButhio), which is stable to trifluoroacetic acid (TFA) but can be selectively deprotected using thiols, such as dithiothreitol or dithioerythritol. Assembly of the peptide chain in solid-phase, followed by a standard TFA deprotection/resin cleavage step, gave the desired Cys(tButhio)-protected basic region ( 1 ) in good yield ( Fig. 2 ). Alkylation of the free thiol with 4′-methylbromo-2,2′:6′,2′′-terpyridine, followed by treatment of the resulting peptide with dithioerythritol produced the desired thiol 3a . In addition, a control peptide ( 3b ), in which the terpyridine is replaced by a 4′-nitroacetophenone chromophore (NAP), was also synthesized. 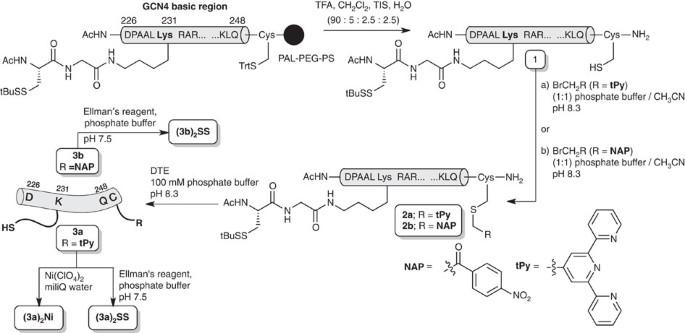Figure 2: Synthesis of the modified monomeric peptides and dimerization reactions. Standard solid-phase peptide synthesis yields the fully protected peptide containing an unprotected C-terminal Cys (1), which is modified in solution to yield the terpyridine derivative (2a) or the nitroacetophenone (NAP) control peptide (2b). Final deprotection of the N-terminal Cys side chain gives the desired bifunctional peptides3aand3b, which can be dimerized as described. The full sequence of the GCN4 basic region peptide is D226PAALKRARNTEAARRSRARKLQ248. Figure 2: Synthesis of the modified monomeric peptides and dimerization reactions. Standard solid-phase peptide synthesis yields the fully protected peptide containing an unprotected C-terminal Cys ( 1 ), which is modified in solution to yield the terpyridine derivative ( 2a ) or the nitroacetophenone (NAP) control peptide ( 2b ). Final deprotection of the N-terminal Cys side chain gives the desired bifunctional peptides 3a and 3b , which can be dimerized as described. The full sequence of the GCN4 basic region peptide is D 226 PAALKRARNTEAARRSRARKLQ 248 . Full size image Monomeric peptides 3a and 3b were dimerized by treatment with DTNB (5,5′-dithiobis-(2-nitrobenzoic acid), Ellman's reagent) in phosphate buffer at pH 7.5. On the other hand, addition of 5 equiv. of Ni(ClO 4 ) 2 to 3a in neutral water promotes the formation of the expected nickel- bis -terpyridine complex, as deduced from liquid chromatography (LC)-mass spectrometry (MS) ( Supplementary Fig. S5 ). DNA-binding studies The DNA-binding properties of the synthetic peptides were studied by electrophoretic mobility shift assays (EMSA) under non-denaturing conditions, and using SYBR-gold for DNA staining. As expected, while monomeric peptide 3a does not bind to short double-stranded (ds)DNAs containing the direct ATF/CREB consensus DNA-binding sequence ( dir : 5′-…ATGA cg TCAT…-3′), addition of 5 equiv. of Ni(ClO 4 ) 2 results in a new slow-migrating band, consistent with the formation of the specific complex between the (3a) 2 Ni dimer and the DNA ( Fig. 3a , lanes 1–3). 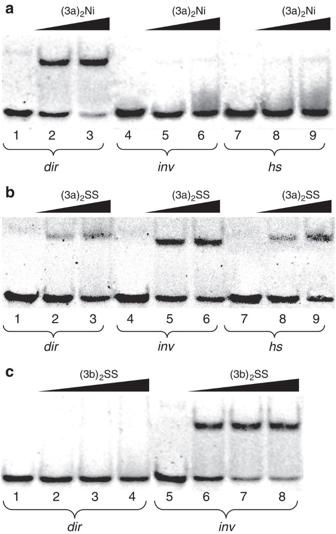Figure 3: EMSA analysis of DNA binding. (a) Lanes 1–3: dsDNAdir(which contains the target ATF/CREB-binding site), lanes 4–6: dsDNAinv(which contains an exchanged binding site), lanes 7–9: dsDNAhs(which contains a consensus half-site). Lanes 2–3, 5–6 and 8–9: 600 and 1200, nM of3aand 5 equiv. of Ni(ClO4)2, as well as excess of TCEP to prevent the oxidation of the thiols. (b) Lanes 1–3: dsDNAdir; lanes 4–6: dsDNAinv; lanes 7–9: dsDNAhs. Lanes 2–3, 5–6 and 8–9: 300 and 600 nM of(3a)2SS. (c) Lanes 1–4: dsDNAdir; lanes 5–8: dsDNAinv. Lanes 2–4 and 6–8: 400, 600, 800 nM of(3b)2SS. The protocol involved addition of peptide solutions in 20 mM Tris-HCl, pH 7.5 to 18 mM Tris-HCl, pH 7.5, 90 mM KCl, 1.8 mM MgCl2, 1.8 mM EDTA, 9% glycerol, 0.11 mgml−1BSA, 2.25% NP-40 and 100 nM of DNA (4 °C, 30 min) and loading into the gel. DNA was detected by fluorescent staining with SYBR-gold. Oligonucleotide sequences (binding sites underlined, only one strand shown):dir: 5′-CGGATGACGTCATTTTTTTTC-3′;inv: 5′-CGGTCATCGATGATTTTTTTC-3′;hs: 5′-CGGATGACG TTCG TTTTTTTC-3′. Figure 3: EMSA analysis of DNA binding. ( a ) Lanes 1–3: dsDNA dir (which contains the target ATF/CREB-binding site), lanes 4–6: dsDNA inv (which contains an exchanged binding site), lanes 7–9: dsDNA hs (which contains a consensus half-site). Lanes 2–3, 5–6 and 8–9: 600 and 1200, nM of 3a and 5 equiv. of Ni(ClO 4 ) 2 , as well as excess of TCEP to prevent the oxidation of the thiols. ( b ) Lanes 1–3: dsDNA dir ; lanes 4–6: dsDNA inv ; lanes 7–9: dsDNA hs . Lanes 2–3, 5–6 and 8–9: 300 and 600 nM of (3a) 2 SS . ( c ) Lanes 1–4: dsDNA dir ; lanes 5–8: dsDNA inv . Lanes 2–4 and 6–8: 400, 600, 800 nM of (3b) 2 SS . The protocol involved addition of peptide solutions in 20 mM Tris-HCl, pH 7.5 to 18 mM Tris-HCl, pH 7.5, 90 mM KCl, 1.8 mM MgCl 2 , 1.8 mM EDTA, 9% glycerol, 0.11 mgml −1 BSA, 2.25% NP-40 and 100 nM of DNA (4 °C, 30 min) and loading into the gel. DNA was detected by fluorescent staining with SYBR-gold. Oligonucleotide sequences (binding sites underlined, only one strand shown): dir : 5′-CGG ATGA CG TCAT TTTTTTTC-3′; inv : 5′-CGG TCAT CG ATGA TTTTTTTC-3′; hs : 5′-CGG ATGA CG TTCG TTTTTTTC-3′. Full size image Importantly, the dsDNA inv , which features an inverted target site (5′-…TCAT cg ATGA…-3′), as well as a control dsDNA containing a single consensus half-site ( hs : 5′-…ATGA cg TTCG…-3′), did not lead to any new bands in the EMSA assays ( Fig. 3a , lanes 4–9). These results demonstrate that the metal-promoted dimers of 3a show a clear preference for binding to the consensus direct site over the inverted alternative. With regard to the N-terminal disulphide dimer (3a) 2 SS , we observed the formation of a DNA complex with its target inverted DNA ( inv , Fig. 3b , lanes 4–6) but, curiously, it also produces retarded bands with the other oligos dir and hs ( Fig. 3b , lanes 1–3, and 7–9). These bands with the non-consensus dsDNAs are more diffuse than those observed with the direct DNA, and most probably arise from a relatively loose complex in which one of the basic regions is interacting specifically in the major groove of the consensus site while the other makes nonspecific contacts [38] . Curiously, the control disulphide (3b) 2 SS , in which the terpyridine was replaced by an inert chromophore, did not elicit such interactions with the non-consensus DNAs ( Fig. 3c ), which suggests that the terpyridine unit might be contributing to the formation of the undesired EMSA bands. Changing the dimerization state Despite the selectivity problem of the N-terminal disulphide dimer, peptide 3a seemed appropriate to explore the viability of controlling site-interactions by altering its dimerization state in the presence of DNA. As expected, reduction of the disulphide bond of (3a) 2 SS by treatment with the reducing agent TCEP (tris(2-carboxyethyl)phosphine) resulted in the formation of monomeric species and hence complete loss of DNA binding to either the direct or the inverse DNA sequence ( Fig. 4 , compare lanes 2 and 6 versus lanes 3 and 7, respectively). Importantly, addition of Ni(ClO 4 ) 2 to the solution obtained after the reduction step generates the C-terminal (3a) 2 Ni dimer, as deduced by the appearance of the corresponding retarded DNA band when incubated with the dsDNA dir ( Fig. 4 , lane 8). This result, which confirms the viability of switching from the disulphide N-terminal dimer to the metal-promoted C-terminal dimer, encouraged us to further refine the design in order to achieve better sequence selectivities. 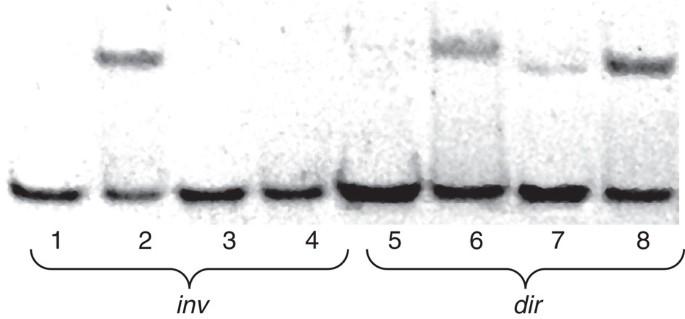Figure 4: EMSA analysis of DNA binding after changing the dimerization state. Two stock solutions of dimeric peptide(3a)2SS(3 μM) in 20 mM Tris-HCl pH 7.5 in the presence 500 nM of either dsDNAsinv(lanes 1–4) ordir(lanes 5–8) were successively treated at room temperature with TCEP (40 mM), 5 min, and Ni(ClO4)2(15 μM) another 5 min. Aliquots of the different solutions, each containing over 50 nM DNA, were mixed with the loading buffer and run under non-denaturing conditions. Lanes 2 and 6:(3a)2SS; lane 3 and 7: same mixture after treatment with TCEP; lanes 4 and 8: previous mixture after treatment with Ni(ClO4)2. DNA was detected by fluorescent staining with SYBR-gold. Figure 4: EMSA analysis of DNA binding after changing the dimerization state. Two stock solutions of dimeric peptide (3a) 2 SS (3 μM) in 20 mM Tris-HCl pH 7.5 in the presence 500 nM of either dsDNAs inv (lanes 1–4) or dir (lanes 5–8) were successively treated at room temperature with TCEP (40 mM), 5 min, and Ni(ClO 4 ) 2 (15 μM) another 5 min. Aliquots of the different solutions, each containing over 50 nM DNA, were mixed with the loading buffer and run under non-denaturing conditions. Lanes 2 and 6: (3a) 2 SS ; lane 3 and 7: same mixture after treatment with TCEP; lanes 4 and 8: previous mixture after treatment with Ni(ClO 4 ) 2 . DNA was detected by fluorescent staining with SYBR-gold. Full size image Optimization of the design As previously shown, in contrast to the result with the terpyridine containing disulphide (3a) 2 SS , the dimer (3b) 2 SS showed very low affinities for the non-consensus DNAs dir and hs , which suggest that the terpyridine group is actively contributing to the weaker, undesired binding mode, probably by providing DNA intercalating capability. Therefore, we decided to use a terpyridine unit featuring two methyl substituents, which might hinder that interaction. To facilitate the synthetic procedures, and minimize solution chemistry, the terpyridine group was introduced on solid-phase on the side chain of a lysine residue engineered at the C-terminal position of the peptide, which also provided for further isolating the terpyridine from the DNA-binding basic region. As shown in Fig. 5 , the synthetic protocol involved removal of the Mtt (4-methyltrityl) protecting from the first Lys side chain under mild acidic conditions [39] , and coupling of 5,5′′-dimethyl-[2,2′:6′,2′′-terpyridine]-4′-carboxylic acid to the resulting amine, followed by introduction of the rest of the peptide sequence. The lysine at position 231 was inserted as Lys(alloc), which allowed the selective deprotection of its side chain by Pd catalysis after acetylation of the N-terminal Asp226 (ref. 40 ). Finally, the Gly-Cys linker was assembled onto the Lys side chain and acetylated to give the full terpyridine-modified peptide attached to the resin. Standard deprotection and cleavage, and high-performance liquid chromatography (HPLC) purification afforded the desired peptide 4 , in an overall 30% yield. This peptide can be readily dimerized upon oxidation with 5,5′-dithiobis-(2-nitrobenzoic acid) (DTNB) in a slightly basic phosphate buffer. On the other hand, addition of Ni 2+ or Fe 2+ salts to peptide 4 led to the formation of the expected bis-terpyridine complexes (4) 2 Ni and (4) 2 Fe , which could be isolated and identified by MS ( Supplementary Figs S10 and S11 ). 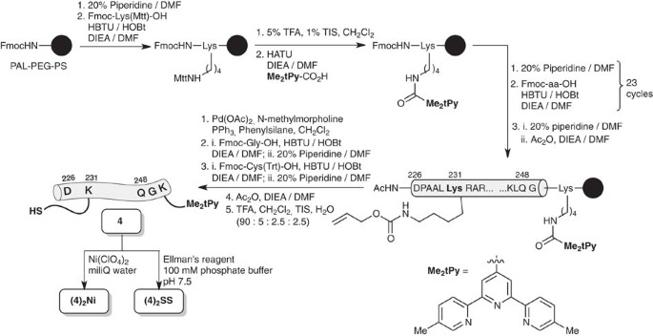Figure 5: Synthesis of peptide 4 and its N and C-terminal dimers. Incorporation of the terpyridine moiety at the C-terminal lysine side chain while the peptide is still bound to the resin. The tether on the lysine 231 is similar to that used in the peptide1(Gly–Cys,Fig. 2). Figure 5: Synthesis of peptide 4 and its N and C-terminal dimers. Incorporation of the terpyridine moiety at the C-terminal lysine side chain while the peptide is still bound to the resin. The tether on the lysine 231 is similar to that used in the peptide 1 (Gly–Cys, Fig. 2 ). Full size image DNA-binding studies with the peptide 4 As shown in the Fig. 6a , the dimer (4) 2 Ni , made in situ by addition of Ni(ClO 4 ) 2 to the peptide 4 , binds the consensus direct DNA dir , but does not give rise to retarded bands with the inverse DNA inv . A titration using a P 32 -labelled ds-oligonucleotide allowed us to calculate an apparent binding constant of ≈299 nM at 4 °C ( Supplementary Fig. S14 ). More importantly, in contrast to the former disulphide (3a) 2 SS , the new N-terminal dimer (4) 2 SS displayed good selectivity for its target sequence (DNA inv ) against the non-consensus dir dsDNA ( Fig. 6b ), although, curiously, in order to observe neat EMSA retarded bands we found that it is important that the binding mixture contains Ni 2+ or Co 2+ metal ions. It is probable that coordination of the metals to either terpyridine, complex observed by MS ( Supplementary Fig. S12 ), might prevent unproductive folding or nonspecific DNA binding, and hence favour the formation of the desired DNA complexes. Remarkably, addition of (NH 4 ) 2 Fe(SO 4 ) 2 to (4) 2 SS suppresses the formation of complexes with the target DNA inv , most probably because of the intrinsic tendency of Fe 2+ to simultaneously bind both terpyridines, thus forming a stable macrocyclic species unable to bind DNA. In the presence of 5 equiv. of Ni(ClO 4 ) 2 , and using radioactive EMSA experiments, we calculated a K D of ≈375 nM for the binding of (4) 2 SS to its consensus inverted DNA inv ( Supplementary Fig. S13 ). 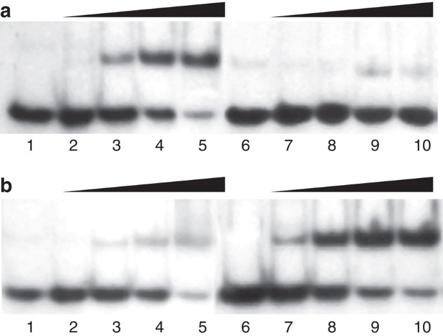Figure 6: Radioactive EMSA analysis of the DNA-binding properties of peptide 4 and its dimeric derivatives. (a) and (b) Lanes 1–5: dsDNAdir(100 nM); lanes 6–10: dsDNAinv(100 nM); a small proportion (~0.1%) of the oligonucleotides are labelled with32P for radioactive detection. (a) Lanes 2–5 and lanes 7–10: 200, 600, 1,000, 1,600 nM of peptide 4 with 5 equiv. of Ni(ClO4)2, and excess of TCEP. (b) Lanes 2–5 and lanes 7–10: 100, 300, 500, 800 nM of peptide(4)2SSin the presence of 5 equiv. of Ni(ClO4)2. Figure 6: Radioactive EMSA analysis of the DNA-binding properties of peptide 4 and its dimeric derivatives. ( a ) and ( b ) Lanes 1–5: dsDNA dir (100 nM); lanes 6–10: dsDNA inv (100 nM); a small proportion (~0.1%) of the oligonucleotides are labelled with 32 P for radioactive detection. ( a ) Lanes 2–5 and lanes 7–10: 200, 600, 1,000, 1,600 nM of peptide 4 with 5 equiv. of Ni(ClO 4 ) 2 , and excess of TCEP. ( b ) Lanes 2–5 and lanes 7–10: 100, 300, 500, 800 nM of peptide (4) 2 SS in the presence of 5 equiv. of Ni(ClO 4 ) 2 . Full size image To get further insights on the performance of the C- and N-terminal dimers, we measured the binding preferences in solution, and in the presence of excess of a competitor DNA (calf-thymus), using fluorescence anisotropy titrations with rhodamine-labelled oligonucleotides ( Fig. 7 ). Thus, a solution of Rhodamine-labelled oligonucleotide dir ( Rho-dir ) was incubated with increasing concentrations of (4) 2 Ni in the presence of a competitive nonspecific calf-thymus DNA (50 μM in base pairs) at 10 °C, and the anisotropy at 585 nm was measured after each addition. We obtained a typical titration profile, which could be fitted to a simple 1:1 binding model with an apparent K D of ≈670 nM. In contrast, incubation of the non-target rhodamine-labelled Rho-inv oligonucleotide under the same conditions with increasing concentrations of this C-terminal dimer resulted in a less pronounced titration curve with a much weaker K D of ≈25 μM. Using similar experiments, we found that (4) 2 SS displays a higher affinity for the consensus rhodamine-labelled inv oligo ( K D ≈758 nM) than for the non-target Rho-dir oligonucleotide ( K D ≈5.3 μM). These values are in agreement with those obtained using radioactive EMSA titrations, and further support the differential binding of the two dimers. The observation of a more intense anisotropy with the two non-target DNAs ( (4) 2 Ni/ Rho-inv and (4) 2 SS/ Rho-dir )), than with the specific complexes ( (4) 2 Ni/ Rho-dir and (4) 2 SS/ Rho-inv ) is consistent with the formation of more compact species in the case of the specific interactions, and larger complexes with the non-target oligonucleotides, which therefore display slower dynamics. 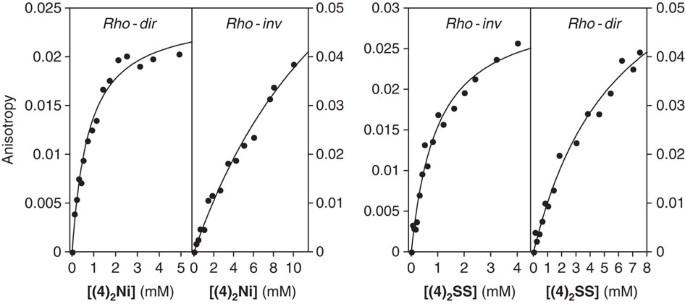Figure 7: Fluorescence anisotropy analysis of the DNA-binding properties of peptide 4 and its dimeric derivatives. Fluorescence anisotropy titrations of the C- and N-terminal dimers with DNA oligonucletotides in 20 mM Tris-HCl, pH 6.5, 100 mM NaCl at 10 °C. Left: 50 nM of rhodamine-labelledRho-dirandRho-involigonucleotides in the presence of 50 μM concentration (in base pairs) of nonspecific calf-thymus DNA, with increasing concentrations of C-terminal(4)2Nidimer (stock solution: 400 μM of 4, 600 μM Ni(ClO4)2and 5 mM of TCEP). Right: 50 nM of rhodamine-labelledRho-dirandRho-involigonucleotides in the presence of nonspecific calf-thymus DNA (50 μM base pairs) with increasing concentrations of N-terminal(4)2SSdimer (stock solution: 200 μM of(4)2SS, 600 μM Ni(ClO4)2). Lines represent best fits to a 1:1 binding model.Rho-inv: Rho-TGGAG TCAT CG ATGA CTCGT-3′;Rho-dir: Rho-TGGAG ATGA CG TCAT CTCGT-3′; excitation at 559 nm and anisotropy measured at 585 nm. Figure 7: Fluorescence anisotropy analysis of the DNA-binding properties of peptide 4 and its dimeric derivatives. Fluorescence anisotropy titrations of the C- and N-terminal dimers with DNA oligonucletotides in 20 mM Tris-HCl, pH 6.5, 100 mM NaCl at 10 °C. Left: 50 nM of rhodamine-labelled Rho- dir and Rho - inv oligonucleotides in the presence of 50 μM concentration (in base pairs) of nonspecific calf-thymus DNA, with increasing concentrations of C-terminal (4) 2 Ni dimer (stock solution: 400 μM of 4, 600 μM Ni(ClO 4 ) 2 and 5 mM of TCEP). Right: 50 nM of rhodamine-labelled Rho - dir and Rho - inv oligonucleotides in the presence of nonspecific calf-thymus DNA (50 μM base pairs) with increasing concentrations of N-terminal (4) 2 SS dimer (stock solution: 200 μM of (4) 2 SS , 600 μM Ni(ClO 4 ) 2 ). Lines represent best fits to a 1:1 binding model. Rho - inv : Rho-TGGAG TCAT CG ATGA CTCGT-3′; Rho - dir : Rho-TGGAG ATGA CG TCAT CTCGT-3′; excitation at 559 nm and anisotropy measured at 585 nm. Full size image Finally, circular dichroism experiments were consistent with the behaviour observed in the EMSA experiments. Thus, incubation of the N-terminal disulphide dimer (4) 2 SS with its target sequence ( DNA inv ) resulted in a significant increase in the negative ellipticity at 222 nm, consistent with the α-helical folding expected for an specific interaction [14] , [41] . This increase is not observed with the natural ATF/CREB sequence contained in the dir oligo; likewise, the C-terminal dimer (4) 2 Ni only showed an increase in the negative ellipticity in the presence of its target dir DNA, but not with the swapped inv DNA (see Supplementary Fig. S17 ). Switching between sites Once we confirmed that peptide 4 exhibits the desired orthogonal DNA binding, we were interested in exploring the viability of a sequence-selective recognition in a situation where both target sites are simultaneously available for binding. Thus, a stock solution containing peptide 4 was added to a 50 nM equimolar mixture of both dsDNAs, containing the direct and the inverse sequences dir1 and inv . Note that in this case we use ds-oligonucleotides of different lengths in order to distinguish the binding to either of them. As anticipated, the monomer by itself is unable to elicit retarded shifts ( Fig. 8a , lane 3); addition of 1 equiv. of Ellman’s reagent (DTNB) and 5 equiv. of Ni(ClO 4 ) 2 to that solution resulted and in the appearance of a new band consistent with the formation of a specific complex with the inverse DNA inv ( Fig. 8a , band a in lane 4, and control lane 1). Interestingly, addition of TCEP to the mixture led to the disappearance of this complex and the formation of a new retarded band involving the oligo dir1 , consistent with the DNA binding of the in situ formed dimer ( 4) 2 Ni ( Fig. 8a , band b in lane 5, and control lane 2). A new addition of DTNB dismounts this complex and regenerates binding to the inverse DNA. Despite the excess of reagents in the mixture, it is yet possible to induce a new switch and regenerate binding to other DNA. These results represent the first proof of concept on the viability of making molecules that can be induced to jump between two different DNA sites, at will, in response to specific external stimuli. 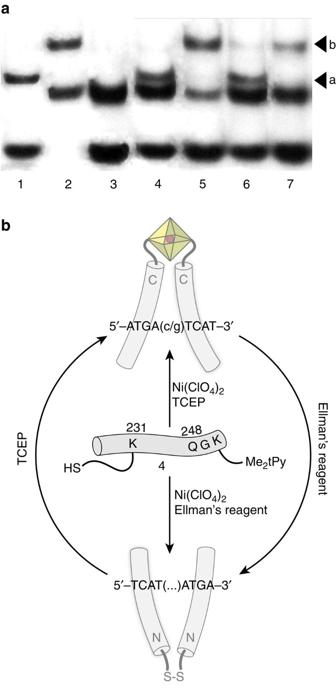Figure 8: Dynamic target DNA selection by peptide 4. (a) Radioactive EMSA experiments: A stock solution containing an equimolar concentration of ds-oligonucleotidesdir1andinv(3 μM, a small proportion of the oligonucleotides are labelled with32P) in the presence of peptide4(36 μM) was successively treated at room temperature with the oxidant (DTNB (0.5 equiv.) and Ni(ClO4)2(5 equiv.)), the reducing agent (TCEP, 40 mM), and again DTNB (40 mM) and TCEP (80 mM); after 2–3 min of reaction, aliquots of the solutions resulting after each step, were mixed with the loading buffer and run under non-denaturing conditions. Lane 1: DNAinv(50 nM) in the presence of 300 nM of(4)2SS; lane 2: DNAdir1(50 nM) in the presence of 600 nM peptide4and Ni(ClO4)2(5 equiv.). Lanes 3–7, aliquots of the above reaction mixtures containing both dsDNAs (~50 nM of each) and peptide4. Lane 3: starting mixture; lane 4: mixture after the first addition of DTNB (and Ni(ClO4)2) lane 5: mixture after the addition of TCEP; lane 6: mixture after the second addition of DTNB; lane 7: mixture after the last addition of TCEP.dir1: 5′-CGGATGACGTCATTTTTTTTCG TTACGAAGGCC-3′. (b) Cartoon representation of the switching process. Figure 8: Dynamic target DNA selection by peptide 4. ( a ) Radioactive EMSA experiments: A stock solution containing an equimolar concentration of ds-oligonucleotides dir1 and inv (3 μM, a small proportion of the oligonucleotides are labelled with 32 P) in the presence of peptide 4 (36 μM) was successively treated at room temperature with the oxidant (DTNB (0.5 equiv.) and Ni(ClO 4 ) 2 (5 equiv. )), the reducing agent (TCEP, 40 mM), and again DTNB (40 mM) and TCEP (80 mM); after 2–3 min of reaction, aliquots of the solutions resulting after each step, were mixed with the loading buffer and run under non-denaturing conditions. Lane 1: DNA inv (50 nM) in the presence of 300 nM of (4) 2 SS ; lane 2: DNA dir1 (50 nM) in the presence of 600 nM peptide 4 and Ni(ClO 4 ) 2 (5 equiv.). Lanes 3–7, aliquots of the above reaction mixtures containing both dsDNAs (~50 nM of each) and peptide 4 . Lane 3: starting mixture; lane 4: mixture after the first addition of DTNB (and Ni(ClO 4 ) 2 ) lane 5: mixture after the addition of TCEP; lane 6: mixture after the second addition of DTNB; lane 7: mixture after the last addition of TCEP. dir1 : 5′-CGG ATGA CG TCAT TTTTTTTCG TTACGAAGGCC-3′. ( b ) Cartoon representation of the switching process. Full size image Recent years have witnessed important advances in the design and preparation of switchable on-off DNA binders. However, molecules that target different DNA sites in response to specific signals, or that can switch between specific DNA sites, have not been developed. Inspired by the concept of combinatorial gene regulation, which is particularly common for bZIP-type of TFs, we have made designed derivatives of bZIP basic regions that can be induced to bind to different DNA sites depending on their dimerization mode. In particular, our results show that installing a suitable terpyridine moiety at the C-terminus of the basic region of GCN4, and a cysteine residue at its N-terminus, it is possible to induce either a C- or N-terminal dimerization by using appropriate triggers. The C-terminal dimerization can be induced by metals like Ni +2 , while the addition of an oxidant, such as Ellman’s reagent, promotes a disulphide dimerization through the N-terminus. The resulting dimers show a more than remarkable selectivity for their cognate-binding sites. Therefore, whereas the C-terminal metallodimer binds the natural ATF/CREB-binding site (5′-ATGA cg TCAT-3′) >40 times better than the swapped sequence (5′-TCAT cg ATGA-3′), the N-terminal disulphide dimer binds the inverted sequence over 10 times better than the ATF/CREB site. The high DNA-binding selectivity of each dimeric state allows the precise targeting of each site in mixtures containing both oligonucleotides or in the presence of an excess of calf-thymus DNA. Importantly, our results indicate that the dimerization can be also triggered in situ , in the presence of DNA. Therefore, the peptide can be driven to either DNA target site by using specific external signals that code its dimerization mode. It is even possible to induce a reversible ‘hopping between sites’ in a stimuli-responsive manner ( Fig. 8b ). This relatively simple design shows many of the features found in natural TFs, namely cooperativity, reversibility, high selectivity and response to specific environmental signals, and thus represent a starting point for the design of more complex DNA combinatorial interaction networks and for gaining a more precise control on the artificial regulation of genes. General All reagents were acquired from commercial sources: dimethyl formamide (DMF) and TFA were purchased from Scharlau, CH 2 Cl 2 from Panreac, CH 3 CN from Merck, [2,2′:6′,2′′-terpyridin]-4′-yl-methanol was purchased from HetCat. The rest of reagents were acquired from Sigma-Aldrich. All peptide synthesis reagents and amino-acid derivatives were purchased from GL Biochem (Shanghai) Ltd and Novabiochem. Amino acids were purchased as protected Fmoc amino acids with the standard side-chain protecting scheme, except for the orthogonally protected Fmoc-Lys(Alloc)-OH and Fmoc-Lys(Mtt)-OH. Reactions were followed by analytical reversed phase (RP)-HPLC with an Agilent 1100 series LC/MS using an Eclipse XDB-C8 analytical columna (4.6 × 150 mm, 5 μm). Electrospray Ionization Mass Spectrometry was performed with an Agilent 1100 Series LC/MSD model in positive scan mode using direct injection of the purified peptide solution into the MS. Standard conditions for analytical RP-HPLC consisted on an isocratic regime during the first 5 min, followed by a linear gradient from 5 to 75% of solvent B for 30 min at a flow rate of 1 ml min −1 (A: water with 0.1% TFA, B: acetonitrile with 0.1% TFA). Compounds were detected by ultraviolet absorption at 220, 270, 304 and 330 nm. Purification were performed by semipreparative RP-HPLC with an Agilent 1100 series LC using a Luna 5u C18(2) 100A (5 μm, 10 × 250 mm) reverse-phase column from Phenomenex. Matrix-assisted laser desorption/ionization mass spectrometry (MS) was performed with a Bruker Autoflex matrix-assisted laser desorption/time-of-flight (TOF) model in positive scan mode by direct irradiation of the matrix-absorbed peptide. Concentrations were measured using the listed extinction coefficients. Calf-thymus DNA was acquired from Sigma-Aldrich. Oligonucleotides were purchased from Thermo Fisher Scientific GmbH on a 0.2 mmol scale as freeze-dried solids. After solving in H 2 O milliQ their concentrations were measured by ultraviolet absorption at 260 nm with a BioRad SmartSpec Plus Spectrophotometer. Absorbance was measured twice and concentrations were calculated applying Lambert-Beer’s equation. The molar extinction coefficients of single-strand oligonucleotides were calculated by using the following formula [42] , ɛ(260 nm)={(8.8 × #T)+(7.3 × #C)+(11.7 × #G)+(15.4 × #A)} × 0.9 · 103 M −1 cm −1 , where #A, #T, #C, #G stand for the number of each type of bases in the DNA strand. The concentration of Rhodamine-labelled oligonucleotides was calculated using the molar extinction of rhodamine. Oligonucleotides were hybridized by mixing complementary sequences at equal molar concentration (50 μM), heating at 90 °C for 10 min and then slowly cooling the mixture to room temperature over 1 h. The synthesis of the terpyridine moieties and their coupling to the peptides is detailed in the Supplementary Methods . Electrophoretic mobility shift assay EMSA were performed with a BioRad Mini Protean gel system, powered by an electrophoresis power supplies PowerPac Basic model, maximum power 150 V, frequency 50.60 Hz at 140 V (constant V). The binding reactions were performed over 30 min in 18 mM Tris (pH 7.0), 50 mM KCl, 1.2 mM MgCl 2 , 0.5 mM EDTA, 9% glycerol, 0.11 mg ml −1 BSA and 4.2% NP−40 at 4 °C. In the experiments analysed by fluorescent staining we used 100 nM of the unlabelled dsDNAs and a total incubation volume of 20 μl. In the experiments with 32 P-labelled DNAs we used ~100 pM of labelled dsDNAs and 100 nM of the same unlabelled dsDNAs in a 20-μl binding mixture. Use of lower amounts of DNA gave less clear gels because of precipitation. In order to prevent the oxidation of peptides with free thiols, 2 mM of TCEP is present in the incubation solution. Products were resolved by polyacrylamide gel electrophoresis using a 10% non-denaturing poliacrylamide gel and 0.5 × TBE buffer, and analysed by autoradiography (when radioactivity was used) or by staining with SyBrGold ( Molecular Probes : 5 μl in 50 ml of 1 × TBE) for 10 min and visualized by fluorescence. The labelling of oligonucleotides with 32 P was accomplished in the following manner: 1 μl of the single-strand oligonucleotide which will be labelled (10 μM), 1 μl kinase buffer 10 × (40 mM, Tris–HCl pH 7.5, 10 mM MgCl 2 , 5 mM dithiothreitol), 2 μl ATP (ATP (ϒ-32P) (5,000 Ci mmol −1 )) and 0.5 μl of the kinase (10 units μl −1 ); after shaking, the mixture is heated for 1 h at 37 °C, and then quenched by heating for 10 min at 95–100 °C. Peptide synthesis C-terminal amide peptides were synthesized following standard peptide protocols (Fmoc/tBu strategy) on a 0.1 mmol scale using a 0.19 mmol g −1 loading Fmoc-PAL-PEG-PS resin from Applied Biosystems, using a PS3 automatic peptide synthesizer from Protein Tecnologies. The amino acids were coupled in fourfold excess using HBTU (O-Benzotriazole- N , N , N ′, N ′-tetramethyl-uronium-hexafluoro-phosphate) as activating agent. Each amino acid was activated for 30 s in DMF before being added onto the resin, and couplings were conducted for 30 min. Deprotection of the temporal Fmoc protecting group was performed by treating the resin with 20% piperidine in DMF for 10 min. Manual couplings were monitored using the TNBS (trinitrobenzene sulphonate) test [43] . The resin cleavage-deprotection was accomplished by shaking the resin-bound peptides for 2 h (~0.025 mmol), in 3 ml of the cleavage cocktail (25 μl of H 2 O, 25 μl of triisopropylsilane, 50 μl of CH 2 Cl 2 and 900 μl of TFA). The resin is filtered, and the TFA filtrate is added to ice-cold diethyl ether (30 ml). After 10 min, the precipitate is centrifuged and washed again with 20 ml of ice-cold ether. The solid residue is dried under argon, dissolved in CH 3 CN/water 1:1 (2 ml) and purified by semipreparative RP-HPLC. The collected fractions are lyophilized and stored at −20 °C. Acetylation of peptides was carried using mixtures of Ac 2 O/DMF (1:2) in the presence of 2 equiv. of DIEA ( N , N -Diisopropylethylamine). Deprotection of Lys(Alloc) side chain The resin-bound peptide (~0.05 mmol) was treated overnight at room temperature with a deoxygenated mixture of methylmorpholine (55 μl, 10 equiv. ), triphenylphosphine (20 mg, 1.5 equiv. ), phenylsilane (62 μl, 10 equiv.) and Pd(OAc) 2 (3.4 mg, 0.3 equiv.) in CH 2 Cl 2 (2.7 ml). The resin was filtered and washed with DMF (2 × 1.5 ml × 2 min), diethyldithiocarbamate (25 mg in 5 ml of DMF, 2 × 1.5 ml × 5 min), DMF (2 × 1.5 ml × 2 min) and CH 2 Cl 2 (2 × 5 ml × 2 min). Deprotecion of Lys(Mtt) side chain The resin-bound peptide (~0.05 mmol) was treated twice with a mixture of TFA (250 μl), triisopropylsilane (50 μl) and CH 2 Cl 2 (4.7 ml) for 5 min. The resin was then filtered and washed with CH 2 Cl 2 (2 × 5 ml × 2 min). General procedure for the obtention of the disulphide dimers The monomeric thiol-containing peptide was dissolved in 100 mM buffer phosphate (pH 7.5) to give an approximate peptide concentration of 2 mM Ellman’s reagent [44] (0.8 mM in acetonitrile, 0.4 equiv.) was added, and the resulting mixture was stirred for 20 min at room temperature. The reaction was quenched using 0.1% aqueous TFA, and the crude purified by RP-HPLC. The collected fractions were lyophilized and stored at –20 °C, after characterization. The dimeric peptides were obtained in yields over 70%. Fluorescence anisotropy Steady-state fluorescence anisotropy measurements were made in a Jobin-Yvon Fluoromax-3 (DataMax 2.20), coupled to a temperature controller Wavelength Electronics LFI-3751, and using a standard Hellma semi-micro cuvette (114F-QS, 10 mm light path). Titrations were carried out at 10 °C using the following parameters: λ ex =559 nm (bandwidth 2.0 nm), λ em =585 nm (bandwidth 12.0 nm), 1 s integration time, and each measure was taken in triplicate. Titrations were made by adding increasing amounts of the desired peptide to a solution containing a rhodamine-labelled oligonucleotide (50 nM) in 20 mM Tris–HCl pH 6.5 100 mM NaCl and 50 μM concentration (in base pairs) of nonspecific calf-thymus DNA. Circular dichroism spectroscopy CD measurements were made in a 2-mm cell at 4 °C. Samples contained 5 μM of corresponding dsDNA (when present) and 5 μM of peptides in 10 mM phosphate buffer (pH 7.5) and 100 mM of NaCl. The CD spectra of the peptides (when measured in the presence of DNA) were calculated as the difference between the spectrum of the peptide/DNA mixture and the measured spectrum of a sample of the DNA oligonucleotide. How to cite this article: Mosquera, J. et al . Stimuli-responsive selection of target DNA sequences by synthetic bZIP peptides. Nat. Commun. 4:1874 doi: 10.1038/ncomms2825 (2013).